Unveiling viral–host interactions within the ‘microbial dark matter’ Viruses control natural microbial communities. Identification of virus–host pairs relies either on their cultivation or on metagenomics and tentative assignment based on genomic signatures. Both approaches have severe drawbacks when aiming to target such pairs within the uncultured majority. Here we present an unambiguous way to assign viruses to hosts that does not rely on any previous information about either of them nor requires their cultivation. First, genomic contents of individual cells present in an environmental sample are retrieved by means of single-cell genomic technologies. Then, individual cell genomes are hybridized against a set of individual viral genomes from the same sample, previously immobilized on a microarray. Infected cells will yield positive hybridization as they carry viral genomes, which can be then sequenced and characterized. Using this method, we pinpoint viruses infecting the ubiquitous hyperhalophilic Nanohaloarchaeota , included in the so-called ‘microbial dark matter’ (the uncultured fraction of the microbial world). Microbes and their viruses constitute the most abundant and diverse group within the biosphere. The interactions among viruses and their microbial hosts have a central influence on biogeochemical cycles, on the control of numbers, diversity and evolution of microbes and even on human health [1] , [2] . However, owing to limitations in the available techniques, there is a lack of knowledge about the interaction patterns between viruses and hosts in natural communities given that their description relies on the identification of viruses, hosts and viral–host ranges [3] . Although this can be readily accomplished for isolated virus–host pairs, it is not technically feasible for uncultured viruses/hosts, which constitute the majority of microbes on the planet. Metagenomic analyses of cellular and viral fractions have provided valuable information on ecologically relevant virus–host interactions, such as in Prochlorococcus , from which previous genomic information was available [4] . However, shotgun metagenomics does not allow for the unambiguous identification of individual virus–host pairs given the limitations of reconstructing individual viral genomes from short read data sets. Cloning of individual viral genomes from environmental samples into fosmids circumvents assembly limitations [5] , [6] , [7] and allows for the tentative assignment of viruses to their hosts based on guanine/cytosine (GC) content and genomic signature comparisons [5] , [6] , [7] , [8] of viral and host genomes. However, although this approach is very useful, it has technical limitations and, in addition, can only be used for assigning viruses to hosts from which genomic information is previously available. Moreover, in the absence of further proof, the assignment remains partly speculative even if complete genomes are recovered, given that there are well-known virus–host pairs with deviant genomic signatures [5] . Recently, Allers et al . [9] have developed a PhageFISH method that detects both replicating and encapsidated (intracellular and extracellular) viral DNA, while simultaneously identifying and quantifying host cells during all stages of infection. For this purpose, probes targeting the viral genome and the small subunit (SSU) rRNA of the microbial host are used. This method offers great possibilities to study virus–microbe interactions in nature and can bridge the gap between metagenomics and direct quantification of viral–host pairs in natural samples. However, it still relies on the previous information of such pairs and cannot distinguish between very close viral genomes or microbial hosts with identical SSU rRNAs. To the best of our knowledge, there are only two previous examples in which viruses have been unambiguously assigned to their uncultured hosts, both using single-cell technologies. In the first case [10] , the sequencing of an individual marine protist revealed the presence of a single-stranded DNA virus infecting the host cell at the time of sampling. This finding illustrates the feasibility of describing virus–host systems by isolation of all individuals present in a sample followed by the sequencing of their genomes. However, this approach would require a considerable sequencing and downstream bioinformatics effort since without any previous information, both infected and uninfected hosts would have to be sequenced and analysed. In the second example [11] , viruses infecting individual cells residing in the termite hindgut were detected by PCR with specific primers for a viral marker gene. However, there are no viral markers present in all viral genomes and thus, either previous information regarding the viruses present in the analysed sample must be available or the search has to be restricted to a group of virus with known markers. Here, to circumvent these limitations, we describe a method that unambiguously assigns viruses to uncultured hosts and does not rely on previous information of any of them nor requires their cultivation. This approach takes advantage of two high throughput techniques that have proven very useful in microbial ecology: single-cell genomics and microarrays. We use this method to detect virus–host pairs in order to investigate virus–microbe infection networks in hypersaline environments. Hypersaline systems harbour the highest densities of viruses reported so far for aquatic samples [12] as well as a diverse assemblage of Bacteria and Archaea, that is often dominated by the square archaeon Haloquadratum walsbyi and contains significant numbers of the recently described Nanohaloarchaeota [13] . The Nanohaloarchaea , along with four other major uncultured prokaryote groups within the unexplored ‘microbial dark matter’, form a monophyletic superphylum called DPANN, for which cultured representatives are not currently available [14] . Here, we target viruses infecting Nanohaloarchaea cells after proving the feasibility of our protocol with the appropriate controls. Overview of the method In short ( Fig. 1 ), individual cells presented in an environmental sample are separated by means of fluorescence-activated cell-sorting, lysed and their genomes amplified by multiple displacement amplification (MDA) [14] , [15] , [16] , [17] , [18] . In parallel, the viral fraction of the sample is concentrated and individual viral genomes are purified and cloned in fosmids, which are immobilized on a microarray (‘virochip’). Then, single-amplified genomes (SAGs) from individual cells are hybridized with the ‘virochip’. If a single cell is infected by a virus at the time of sampling, then its SAG would yield a hybridization signal with the ‘virochip’ (provided that the corresponding virus has been cloned). Further sequencing analysis of the SAG and the corresponding cloned viral genome would allow for the identification of both of them and confirm the presence in the sample of such virus–host pair. This approach can be used to look for viruses infecting specific groups of prokaryotes or even to target eukaryotic cells. For these purposes, targeted SAGs could be identified before hybridization by means of, for instance, SSU rRNA gene sequencing. 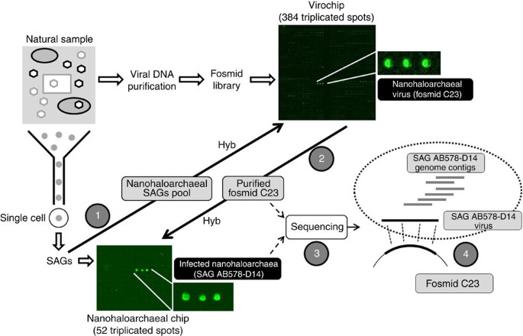Figure 1: Experimental design used to assign viruses to hosts in natural assemblages. Water samples from a crystallizer pond were used for cell sorting and virus concentration. Viral DNA was purified and cloned in fosmids, which were immobilized in the ‘virochip’. Single-amplified genomes (SAGs) identified asNanohaloarchaeawere pooled and hybridized against the ‘virochip’ yielding a high signal with fosmid C23 (1). Fosmid C23 was purified and hybridized against a new chip containing the 52 nanohaloarchaeal SAGs (the ‘Nanohaloarchaeal chip’) (2). A strong hybridization signal was observed in the position of SAG AB578-D14. Both the fosmid C23 and the SAG AB578-D14 were further sequenced and analysed (3, 4). Figure 1: Experimental design used to assign viruses to hosts in natural assemblages. Water samples from a crystallizer pond were used for cell sorting and virus concentration. Viral DNA was purified and cloned in fosmids, which were immobilized in the ‘virochip’. Single-amplified genomes (SAGs) identified as Nanohaloarchaea were pooled and hybridized against the ‘virochip’ yielding a high signal with fosmid C23 (1). Fosmid C23 was purified and hybridized against a new chip containing the 52 nanohaloarchaeal SAGs (the ‘Nanohaloarchaeal chip’) (2). A strong hybridization signal was observed in the position of SAG AB578-D14. Both the fosmid C23 and the SAG AB578-D14 were further sequenced and analysed (3, 4). Full size image Microarray construction, SAG isolation and hybridization Before carrying out the experiments described below, control microarrays were constructed and hybridized as described in the Methods section and in Supplementary Fig. 1 . Samples were taken from crystallizer pond CR30 of Bras del Port solar salterns (Santa Pola, Spain), which has been extensively studied by a vast array of microbial ecology techniques [19] . A 50-μl sample was used for single-cell sorting, generating a total of 936 SAGs that were screened for the 16S rRNA gene for identification. A total of 52 SAGs corresponded to Nanohaloarchaea ( Supplementary Fig. 2 ) and were used for further analysis. In parallel, individual haloviral genomes present in 2 l of the same sample were purified, cloned in fosmids and used for the construction of the ‘virochip’. Fosmids were selected as cloning vectors because they are kept as single copy in the Escherichia coli cells, thus minimizing biases against unstable inserts and increasing the cloning efficiency of haloviral genomes. Besides, the optimum insert size for fosmids (that is, between 30 and 45 kb) corresponds to the size of most haloviral genomes detected in CR30 (ref. 12 ). The ‘virochip’, containing a total of 384 haloviral genomes, was hybridized with the pooled genomes of the 52 nanohaloarchaeal SAGs. As shown in Fig. 1 , one of the fosmids (fosmid C23) yielded a strong hybridization signal. Characterization of a nanohaloarchaeon–virus pair To ascertain which of the Nanohaloarchaea was infected with the cloned virus, a new microarray (‘Nanohaloarchaeal chip’) was constructed with the 52 individual genomes ( Fig. 1 ) and hybridized against the purified fosmid C23. Finally, the tentative virus-containing SAG AB578-D14 (henceforth named as D14) and the fosmid insert were sequenced ( Supplementary Table 1 ). Sequencing indicated that the fosmid insert (of around 30 kb) contained a concatamer of three units of the viral genome. Concatamerization is frequently observed in pulsed field gel electrophoresis preparations of viral genomes with cohesive ends [20] . The size of the repeated unit, that is, the cloned haloviral genome, was 10,021 bp. As expected, the SAG contained the cloned viral genome ( Fig. 2a ), indicating that indeed the nanohaloarchaeon D14 was infected at the time of sampling with the cloned virus (we will refer to this virus as ‘nanohaloarchaeal virus 1’, NHV-1). This was further supported by sequencing data that showed that 99.8% of the recovered viral genome from the host D14 was identical to the viral genome cloned in the fosmid and immobilized in the ‘virochip’ ( Fig. 2a ). In spite of that high level of similarity between both viral genomes (one intracellular, contained within the host D14, and one extracellular, immobilized in the ‘virochip’), a 45-bp region located at the open-reading frame (ORF) 8 ( Table 1 ) displayed 11 single-nucleotide polymorphisms (SNPs) resulting in three non-synonymous substitutions ( Fig. 2 and Supplementary Fig. 3 ). These two genomes could thus correspond to two different virotypes that would be co-occurring in the viral assemblage at the time of sampling. In the case of viruses, a single SNP can impact severely on viral fitness, increasing for instance the adhesion to the host and infection [21] , [22] . Genome annotation ( Table 1 ) showed, although NHV-1 lacked definable capsid genes, that most of the viral ORFs coded for hypothetical conserved proteins related to other uncultured haloviruses characterized in previous studies [5] , [6] , [7] . The lack of integrases (together with the absence of sequence reads overlapping viral and host genomes) suggests a potential lack of lysogenic cycle in NHV-1. In addition, the virus possessed a DNA primase and a viral terminase as well as a putative arsenical resistance repressor-like gene (ORF 7; named as asr R). Interestingly, the catalytic domain of this asrR -like was highly recruited in different geographically distant viral metagenomes ( Fig. 2b ) and also in a previously described cellular metagenome of the same crystallizer CR30 (ref. 19 ); identities 77–100%; Fig. 2b ). 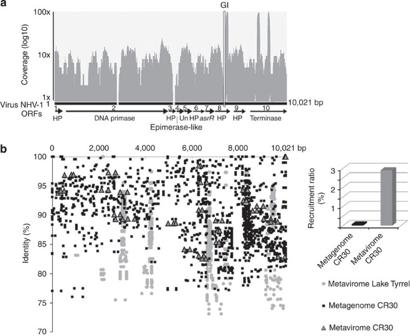Figure 2: Virus NHV-1 infecting nanohaloarchaeon host D14. (a) Mapping of reads from the sequenced host D14 onto the cloned viral genome. A ≥99% of identity threshold and ≥50 bp read length was used. The near complete viral genome was recovered and reconstructed from the infected cell D14. The gap at ORF 8 (nucleotide positions 7,300–7,344) indicates a region of high variability (named as GI) as matched reads displayed an average identity of 77% and a total of 11 SNPs were detected (Supplementary Fig. 3). Three more SNPs at positions 7,401, 8,772 and 9,288 are indicated with white arrows. Gaps at ORFs 2 and 3 (178 bp) are likely due to a bias of the MDA reaction as no reads were found to match with the cloned viral genome. Hypothetical and unknown ORFs are indicated as ‘HP’ and ‘UN’, respectively. (b) Metagenomic fragment recruitment of NHV-1 genome to cellular and viral metagenomes. Data of prokaryote and viral metagenomes from crystallizer CR30 are from Ghaiet al.19and Santoset al.7, respectively. Percentage of recruited reads (parameters as follows: -e-value=0.001, -perc_identity 60) in the metagenome is depicted in the inner panel. Deep Illumina metavirome sequencing data from Lake Tyrrell (Australia) were from Narasingaraoet al.18(NCBI Bioproject accession codePRJNA81851). Furthermore, similar asrR -like sequences were also found ( Supplementary Table 2 ) in several prokaryote genome contigs from the hypersaline Lake Tyrrell [23] , where Nanohaloharchaea were predominant [13] . Arsenic compounds in hypersaline waters are highly prevalent and toxic for organisms, although prokaryotes have evolved different strategies to detoxify or exploit them [24] . Whether the viral asrR -like gene is indeed involved is arsenic metabolism or in other transcriptional regulatory pathways requires further attention. However, it resembled other asrR -like genes detected in prokaryote genomes and metagenomes, which suggests a trans-acting regulator with a conserved role in viral fitness. It is also worth noting that the highest recruited NHV-1 genomic region (intergenic space of ORFs 9 and 10) with the cellular metagenome from crystallizer CR30 ( Fig. 2 ) was similar to sequences of the plasmid PL47 of Hqr. walsbyi of viral origin [25] and a genomic region between the CRISPR 3 and the insertion element protein (IS2) of that very abundant square archaeon. Figure 2: Virus NHV-1 infecting nanohaloarchaeon host D14. ( a ) Mapping of reads from the sequenced host D14 onto the cloned viral genome. A ≥99% of identity threshold and ≥50 bp read length was used. The near complete viral genome was recovered and reconstructed from the infected cell D14. The gap at ORF 8 (nucleotide positions 7,300–7,344) indicates a region of high variability (named as GI) as matched reads displayed an average identity of 77% and a total of 11 SNPs were detected ( Supplementary Fig. 3 ). Three more SNPs at positions 7,401, 8,772 and 9,288 are indicated with white arrows. Gaps at ORFs 2 and 3 (178 bp) are likely due to a bias of the MDA reaction as no reads were found to match with the cloned viral genome. Hypothetical and unknown ORFs are indicated as ‘HP’ and ‘UN’, respectively. ( b ) Metagenomic fragment recruitment of NHV-1 genome to cellular and viral metagenomes. Data of prokaryote and viral metagenomes from crystallizer CR30 are from Ghai et al . [19] and Santos et al . [7] , respectively. Percentage of recruited reads (parameters as follows: -e-value=0.001, -perc_identity 60) in the metagenome is depicted in the inner panel. Deep Illumina metavirome sequencing data from Lake Tyrrell (Australia) were from Narasingarao et al . [18] (NCBI Bioproject accession code PRJNA81851 ). Full size image Table 1 Genome annotation of NHV-1, which infects nanohaloarchaeon AB 578-D14. Full size table Small cell and genome sizes have been predicted as unifying features of the DPANN phyla [14] . 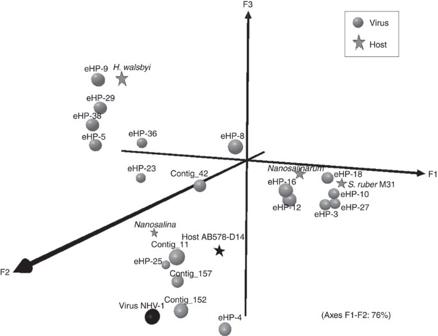Figure 3: Principal component analyses (PCAs) of the dinucleotide frequency signatures of viruses and hosts. Frequency of dinucleotide signatures was calculated and plotted in a PCA plot for reference halophilic prokaryote genomes, the pair NHV-1-Nanohaloarchaeon host D14 and the viral contigs from environmental uncultured halophages (‘eHP-number’ and ‘Contig_number’) from García-Herediaet al.5and Santoset al.7, respectively. Viral and host genomes are represented by spheres and stars, respectively. A total of 51 genomes were included in the PCA plot (see Methods), but for convenience, only selected viruses from same group clustering with its putative host were displayed. Axes F1 and F2 explain 76% of the variance between the analysed genomes. The assembly of the host genome SAG D14 (~1 Mbp; Supplementary Table 3 , Supplementary Fig. 4 ) was similar to that reported for its closest relative Candidatus Nanosalinarum sp. J07AB56 (ref. 13 ) and in the range of Nanohaloarchaeota group [14] . Genome comparison showed that although both Nanohaloarchaea shared a high 16S rRNA gene sequence identity ( Supplementary Fig. 2 ), their genomic content was considerably different ( Supplementary Fig. 5 ). However, in both genomes, most genes coded for hypothetical proteins, many of which were shared by both nanohaloarchaea and present in the corresponding CR30 cellular metagenome [19] ( Supplementary Figs 6–9 and Supplementary Data 1 ). As discussed above, GC content and oligonucleotide frequency signatures have been used to tentatively assign viruses to hosts in natural assemblages without previous cultivation [5] , [7] . In our case, NHV-1 and its nanohaloarchaeon D14 host possessed similar GC content (49% and 51%, respectively). Principal component analysis of dinucleotide frequencies ( Fig. 3 ) revealed that NHV-1 genome grouped with the genomes of the nanohaloarchaeon D14 host and Candidatus Nanosalina ( Fig. 3 ), and also with viral contigs from the above-mentioned CR30 viral metagomic library [7] , which resulted as best BLAST hits for several ORFs of virus NVH-1 ( Table 1 ). Similar results were obtained when tetranucleotide frequency signatures were considered for the analysis ( Supplementary Fig. 9 ). Remarkably, the environmental haloviruses eHP-4 and eHP-25, previously assigned to Nanohaloarchaea hosts according to their codon usage [5] , also clustered with NHV-1. Thus, our data validate the previous assignments of (uncultured) viruses to hosts in hypersaline systems based on genomic signature analyses. Figure 3: Principal component analyses (PCAs) of the dinucleotide frequency signatures of viruses and hosts. Frequency of dinucleotide signatures was calculated and plotted in a PCA plot for reference halophilic prokaryote genomes, the pair NHV-1-Nanohaloarchaeon host D14 and the viral contigs from environmental uncultured halophages (‘eHP- number ’ and ‘Contig_ number ’) from García-Heredia et al . [5] and Santos et al . [7] , respectively. Viral and host genomes are represented by spheres and stars, respectively. A total of 51 genomes were included in the PCA plot (see Methods), but for convenience, only selected viruses from same group clustering with its putative host were displayed. Axes F1 and F2 explain 76% of the variance between the analysed genomes. Full size image Overall, the method presented here can be accommodated within different workflows either to target a specific host group (as done here with the Nanohaloarchaea ) following a wider metagenomic approach or as a tool for discovery of novel viral–host pairs without choosing any specific host. The feasibility of any such untargeted approach would depend, however, on the diversity of the system being analysed since, as is the case with metagenomics, more diverse systems would require greater efforts in terms of microarray construction and recovery of SAGs. Furthermore, although our approach has been used to target double-stranded DNA viral assemblages, modifications can be introduced to make it suitable for double-stranded DNA genomes with covalently bound terminal proteins, single-stranded DNA or even RNA viruses [26] . In addition, the induction of temperate viruses (by means of, for instance, mitomycin C treatment), before applying this method, can provide accession to the dormant virus fraction. One possible limitation of the technique presented here that could mislead the assignment of the virus–host pair is the co-sorting of a cell with a free virus. However, the single-cell sorting mode used here will sort a drop when it contains only one cell in its centre and no other detectable free particles in the drop [27] , which makes the co-sorting of a cell with a virus very unlikely. Other potential limitations of the technique are the co-sorting of the host cell with unspecific viruses attached to it or with free viruses placed in its shade, known in flow cytometry as ‘swarm’ detection [28] . However, our microarray hybridization data does not indicate contamination with free viruses, suggesting an insignificant contribution of ‘swarm’ detection during cell sorting. Nevertheless, a simple pre-enrichment step to remove most free viruses could be routinely implemented before sorting, if needed. In the case of unspecific attached viruses, our data does not support that hypothesis but rather confirms previous assignment data [5] . Here, we have provided a tool that can be used to analyse virus–microbe infection networks over any range of spatiotemporal scales and to draw valuable information on the evolution of virus genomes and the co-evolution with their hosts. This approach can be used to assign viruses to hosts even without previous information about either of them, which makes it suitable for the exploration of microbial dark matter. Sample collection A 50-μl water sample from CR30, a crystallizer pond of Bras del Port salterns (Santa Pola, Spain, 38°12′N, 0°36′W) taken in June 2011 was used for single-cell sorting. The salinity of the sample was 37.2% and harboured 1.74 × 10 7 cells per ml. Cell counting was performed after 4′,6-diamidino-2-phenylindole-dihydrochloride staining (1 μg ml −1 ; Sigma) in an epifluorescence microscope (Leica, type DM4000B; Vashaw Scientifics Inc.). Two liters of the same sample were used for viral DNA extraction. Single-cell sorting and analyses Replicate water samples for single-cell analyses were diluted to 10 5 cells per ml, cryopreserved with 6% glycine betaine (Sigma-Aldrich) and shipped at −20 °C to Single Cell Genomics Center (Maine, USA). For prokaryote detection, diluted subsamples (1 ml) were incubated for 10–120 min with SYTO-9 DNA stain (5 μM final concentration; Invitrogen). The high-nucleic acid cell fraction was targeted for fluorescence-activated cell sorting with a MoFlo (Beckman Coulter) flow cytometer using a 488-nm argon laser for excitation, a 70-μm nozzle orifice and a CyClone robotic arm for droplet deposition into microplates. The cytometer was triggered on side scatter. The ‘single 1 drop’ mode was used for maximal sort purity, which ensures the absence of non-target particles within the target cell drop and the drops immediately surrounding the cell. Single-cell sorting, whole-genome amplification, real-time PCR screens of 16S rRNA genes and sequencing of PCR products were performed at the Bigelow Laboratory Single Cell Genomics Center ( https://scgc.bigelow.org/ ), as described in detail elsewhere [14] , [15] , [16] , [17] , [18] . In brief, individual cells stained with SYTO-9 were sorted using a MoFlo (Beckman Coulter) flow cytometer using a 488-nm argon laser for excitation and a CyClone robotic arm for droplet deposition into microplates. Single cells were then lysed using cold KOH and subjected to whole-genome MDA. The MDA products were diluted 50-fold in sterile TE buffer, and 0.5 μl aliquots of the dilute MDA products served as templates in 5 μl real-time PCR screens for 16S rRNA gene. The partial 16S rRNA gene sequences obtained from nanohaloarchaeon SAGs (~500 bp sequence length) were carefully edited and then aligned using the SILVA aligner ( http://www.arb-silva.de/ ). Only sequences displaying ≥80% of the alignment quality score in the SILVA aligner were considered for the analysis. The alignment was imported into the Geneious R6.1 bioinformatic package (Biomatters Ltd.) and phylogenetic analysis based on neighbour-joining and maximum likelihood (1,000 bootstrap replications) was performed. Viral DNA purification and fosmid library Two liters of the CR30 water sample were centrifuged at 30,000 g (30 min, 20 °C; Avanti J-30I, Beckman). The supernatant was then tangentially filtered through a 30,000 molecular-weight-cutoff Vivaflow filtre cassette (Sartorius Stedim Biotech) and concentrated to 20 ml. Water concentrates were filtered to remove non-centrifuged cells using 0.2 μm filtres (GV Durapore, Millipore) and viruses were then ultracentrifuged at 186,000 g during 2 h at 20 °C in an Optima MAX-XP Ultracentrifuge with the TLA-S5 rotor (Beckman Coulter) and re-suspended in 0.5 ml of 25% sea water (SW), containing (in grams per litre): NaBr, 0.65; NaHCO 3 , 0.17; KCl, 5; CaCl 2 , 0.72; MgSO 4 7H 2 O, 49.49; MgCl 2 6H 2 O, 34.57; NaCl, 195. Halovirus concentrates were mixed with equal volumes of 1.6% low-melting-point agarose (Pronadisa), dispensed into 100-μl moulds, and allowed to solidify at 4 °C. Agarose plugs were incubated for 90 min with 5 μl of Turbo DNA- free kit (Ambion) to digest dissolved DNA (according to the manufacturer’s protocol, 2–3 μl of Turbo DNase digest up to 500 μg ml −1 of DNA in 30 min). The plugs were then incubated overnight at 50 °C in ESP (0.5 M EDTA, pH 9.0; 1% N -laurylsarcosine; 1 mg ml −1 proteinase K) for digestion of DNase and viral capsids. For DNA extraction, plugs were washed with TE-Pefabloc (10 mMTris-HCl, pH 8.0; 1 mM EDTA, pH 8.0; 3 mM Pefabloc, Roche) to inactivate the proteinase K and incubated at 65 °C for 15 min. The mixture of viral DNA and melted agarose was treated with β-agarase (New England BioLabs) for 1.5 h at 42 °C (1 enzyme unit per 0.1 g of melted mixture) and DNA was finally purified using MicroconYM-100 centrifugal filtre devices (Millipore). DNA quality was checked by electrophoresis and its concentration determined by Nanodrop (Thermo Fisher Scientific Inc.). Around 1.5 μg of viral DNA were end-repaired and cloned into pCC2FOS vector using the CopyControl HTP Fosmid Library Production Kit (Epicentre) according to the manufacturer’s recommendations. The EPI300-T1 R strain of E. coli (Epicentre) was used as plating strain. The Fosmid Library Production Kit packages optimally into lambda phage heads inserts with sizes ranging from 30 and 45 kb. All the clones were transferred to four 96-well plates (ABgene), grown with shaking (180 r.p.m.) at 37 °C in LB medium supplemented with 0.2% maltose, 12.5 μg ml −1 of chloramphenicol and 0.5% glycerol, and stored at −80 °C until use. Construction of the ‘control microarray’ and hybridization controls For the experimental controls, genomic DNA from the strain M8 of the extremely halophilic bacterium Salinibacter ruber and a fosmid containing the virus ΦM8-CR4 (which infects M8; Villamor et al ., unpublished) as the insert, were used as the ‘probes’ to be spotted in the ‘control microarray’ ( Supplementary Fig. 1a ). Probe-DNAs were dried using a centrifugal evaporator and re-suspended in microSpotting Solution Plus 1X (Arrayit Corp.) to yield five different concentrations: 10, 50, 100, 250 and 500 ng μl −1 . Spotting was performed with the MicroGrid-TAS II Arrayer (Genomics Solutions) at 22 °C and 50–50% relative humidity on epoxy-substrate slides (Arrayit Corp.) according to the manufacturer’s protocol. Each one of the DNAs used as probes was spotted five times. On the other hand, total DNA from cultures of: (i) non-infected M8 strain and (ii) strain M8 infected with virus ΦM8-CR4 were used as the ‘targets’. DNA from S. ruber cultures was extracted with the DNeasy Blood and Tissue Kit (QIAGEN) according to the manufacturer’s recommendations. For the extraction of the fosmid with the virus ΦM8-CR4, the corresponding clone was grown in 5 ml of terrific broth (TB) medium containing 0.2% maltose, 12.5 μg ml −1 of chloramphenicol and the CopyControl Induction Solution (Epicentre) and the fosmid was extracted using the FosmidMAX DNA Purification Kit (Epicentre), following the protocol supplied. For the labelling of the targets, 4 μg of each DNA were re-suspended in 30 μl of TE (10 mM Tris–HCl pH 8.0, 1 mM EDTA pH 8.0) and treated by sonication with a 2-inch diameter cup horn for Branson ultrasonic cell disruptor (Emerson Electric Co) during 30 s at 70% pulsing. Five hundred nanograms of the sheared DNA were electrophoresed in 1% low electroendosmosis (LE) agarose gels using a 1-kb DNA ladder (Fermentas) as a molecular marker to corroborate that most of the DNA fragments ranged from 0.4 to 1.6 kb. The rest of the sheared DNA was labelled using Cy3-labelled dCTP, random hexamers, the mixture of dNTPs (0.8 mM dATP, dTTP, dGTP; 0.5 mM dCTP) and 50 units of Klenow Fragment (New England Biolabs) for 2 h at 37 °C in a final reaction volume of 50 μl. Three micrograms of Cy3-labelled DNA from (i) the culture of non-infected S. ruber M8 and (ii) the culture of S. ruber M8 infected with virus ΦM8-CR4 were used as the ‘targets’ for the hybridization against the ‘control microarray’ ( Supplementary Fig. 1a ). When labelled DNA from non-infected S. ruber was used as the target, hybridization signals were only positive against the probes where genomic DNA from the strain M8 was spotted ( Supplementary Fig. 1b ). When labelled DNA from the culture of the strain M8 of S. ruber infected with virus ΦM8-CR4 was used as the target, a hybridization signal was observed in all the spots from the ‘control microarray’, demonstrating that the approach was useful for the detection of viruses inside infected cells ( Supplementary Fig. 1c ). Viral microarray (‘virochip’) The 384 clones from the viral fosmid library were grown individually in 1.6 ml of TB medium containing 0.2% maltose, 12.5 μg ml −1 of chloramphenicol and the inducer CopyControl Induction Solution (Epicentre). Fosmids were then extracted using the Perfectprep Plasmid 96 Vac DB kit (Eppendorf) according to the manufacturer’s recommendations and eluting the DNAs twice in 40+40 μl of MilliQ water pre-warmed at 70 °C. Twenty randomly chosen fosmids were analysed by electrophoresis to confirm that they carried inserts with the expected sizes. Fosmids were then transferred to one 384-well plate, dried using a centrifugal evaporator, re-suspended in microSpotting Solution Plus 1X (Arrayit Corp.) yielding ~70 ng μl −1 , and finally spotted on epoxy-substrate slides (Arrayit Corp.) as explained above to obtain the ‘viral microarray’. In addition, PCR products from the 16S rRNA genes of Hqr. walsbyi and S. ruber were also spotted in the ‘virochip’ in order to co-relate fluorescence signals to specific hybridizations (see below). Each one of the DNAs used as probes was spotted three times. As the targets for the corresponding hybridization with the ‘viral microarray’, the 52 SAGs identified as Nanohaloarchaea were used. For this purpose, the 52 nanohaloarchaeal DNAs were pooled and 4 μg were re-suspended in 30 μl of TE (10 mM Tris–HCl pH 8.0, 1 mM EDTA pH 8.0) and treated by sonication with a 2-inch diameter cup horn for Branson ultrasonic cell disruptor (Emerson Electric Co.) during 30 s at 70% pulsing. Five hundred nanograms of the sheared DNA were electrophoresed in 1% LE agarose gels using a 1-kb DNA ladder (Fermentas) as a molecular marker to corroborate that most of the DNA fragments ranged from 0.4 to 1.6 kb. The rest of the sheared DNA were labelled using Cy3-labelled dCTP, random hexamers, the mixture of dNTPs (0.8 mM dATP, dTTP, dGTP; 0.5 mM dCTP) and 50 units of Klenow Fragment (New England Biolabs) for 2 h at 37 °C in a final reaction volume of 50 μl. After hybridization (see below), a clearly strong signal was detected with the virus-containing fosmid C23 ( Fig. 1 ). The ‘signal-to-noise-ratio’ (SNR, a parameter which relates fluorescence intensities with the fluorescence of the background after normalization) in the corresponding C23 spots showed values above 9. To corroborate that these SNR values were in concordance with a specific hybridization signal, labelled DNAs of some SAGs identified as Hqr. walsbyi and S. ruber were also hybridized against the ‘virochip’. In these hybridizations, SNR values in the spots containing the Hqr. walsbyi and S. ruber 16S rRNA genes (that are supposed to reflect specific hybridizations) were always above 5. On the other hand, SNRs between nanohaloarchaeal DNAs and the 16S rRNA genes of Hqr. walsbyi and S. ruber (considered as unspecific hybridizations) showed values below 2 (identity percentages between the 16S rRNA gene sequences of nanohaloarchaea and those from Hqr. walsbyi and S. ruber are below 80%). Nanohaloarchaeal chip The DNAs from the 52 SAGs identified as Nanohaloarchaea were dried, re-suspended in microSpotting Solution Plus 1X (Arrayit Corp.) yielding ~100 ng μl −1 and used as ‘probes’. The obtained ‘Nanohaloarchaeal chip’ was then hybridized against fosmid C23 as the ‘target’. For the purification of the fosmid C23, the corresponding clone was grown in 5 ml of TB medium containing 0.2% maltose, 12.5 μg ml −1 of chloramphenicol and the CopyControl Induction Solution (Epicentre) and the fosmid was extracted using the FosmidMAX DNA Purification Kit (Epicentre). For the labelling, 2.8 μg were treated as described above. Hybridization (see below) yielded a unique signal with the spots corresponding to the nanohaloarchaeal SAG AB578-D14 ( Fig. 1 ). In all the hybridization reactions, printed microarrays were first denatured and pre-hybridized at 42 °C in a pre-hybridization buffer, as previously described by Park and co-workers [29] and then hybridized against ~50 pmol of Cy3-labelled targets. Hybridized arrays were scanned for Cy3 dye in a GenePix 4100A Scanner (Axon Instruments Inc.). The scanned images were saved as 16-bit greyscale-tagged image file format and analysed by quantifying the fluorescence intensity of each spot, using GenePix Pro v.6.0 software (Axon Instruments Inc.). The local background signal was subtracted automatically from the hybridization signal for each spot. Microarray hybridization results were analysed with Genepix pro v.6.0 software (Axon Instruments Inc.). Viral fosmid and SAG AB578-D14 sequencing and assembly SAG AB578-D14 and the corresponding fosmid C23 with the viral insert yielding positive hybridization in the microarray experiment were sequenced using IlluminaMiSeq technology at the Genomic and Bioinformatic Services of the Autonomous University of Barcelona. Paired-end read libraries for Illumina sequencing were prepared with Nextera DNA Sample Preparation Kit according to manufacturer’s protocol, in which 50 ng of DNA template was simultaneously fragmented and tagged with sequencing adapters in a single step. Then, sequencing was performed in a MiSeq Benchtop Sequencer (500 cycles run) generating 2.13 and 1.58 Gb for the fosmid and the SAG D14, respectively ( Supplementary Table 2 ). Assembly of viral genome cloned in the CopyControl HTP Fosmid (Epicentre) was performed with the aid of the previously known sequence of the vector CopyControl pCC2FOS by using Geneious Read Mapper 6.0.3 implemented in Geneious R6.1 (ref. 30 ). First, vector was linearized, and sequences of vector ends, where viral genome insert was cloned, were used as reference scaffold to drive and manage the assembly towards the viral insert. Then a single file with the paired reads was set and used as a query for the mapping-driven assembly with the following parameters: 99% minimum overlap identity, 1% maximum mismatches per read, 100 bp minimum overlap read length, no allowed gaps between two matched reads, 18 word length reads (minimum number of consecutive bases that must match perfectly to find a match between two reads). A total of five iteration mappings was carried out, where reads were mapped to the consensus from the previous iteration. Finally, the resulting consensus sequence from that previous mapping event was used as a reference to span and complete the viral genome with same parameters but using 100 iteration mapping steps instead. Manual inspection was carefully carried out to detected potential misaligned mapping reads or artefacts during the mapping-driven assembly. SAG D14 assembly was performed by three independent strategies that were compared afterwards. In the first strategy, paired reads were merged with FLASH algorithm to extend the length of short reads by overlapping paired-ends reads in order to improve the assembly [31] . When FLASH is used to extend reads before assembly for Illumina data, the resulting assemblies had substantially greater N50 lengths for both contigs and scaffolds. When stringent parameters were used (–m 25, −x 0.2 –M 150; rest parameters by default), 91% of reads were merged and overlapped. Then, merged reads were assembled with the publicly available meta-assembler developed by CAMERA [32] and the resulting contigs were finally assembled in Geneious R6.1 (Biomatters Ltd) if overlapping identity and length was ≥95% and 100 bp, respectively. The second strategy was carried out with VELVET de novo assembler [33] . In doing so, VelvetOptimiser ( http://bioinformatics.net.au/software.velvetoptimiser.shtml ) was initially used to test the optimal parameters for our data that were further used for the assembly. Finally, the new assembler SPAdes [34] specifically designed for sequencing data from SAGs, which outperformed the assembler VELVET-SC for single-cell genomes [35] , was used with the recommended parameters (‘spades.py --sc –k 21,33,55,77,99,127’). Assembly data clearly demonstrate that SPAdes was the best strategy for the genome assembly of the nanohaloarchaeon D14 single cell ( Supplementary Table 3 ). Genome annotation ORFs of viral genome were detected by using the heuristic approach with GenMark Hidden Markov model [36] and annotated by using a combination of BLAST, UNI-PROT BLAST and Conserved-Domain BLAST for the search of functional domains in viral proteins [37] . SAG D14 genome was annotated by using the SEED subsystem publicly available at RAST server [38] and the bioinformatics resources of the US Department of Energy Joint Genome Institute ( http://www.jgi.doe.gov/ ) with the pipeline annotation Prodigal [39] . Metagenome recruitment and genome analysis The basic approach of Rusch et al . [40] was used to estimate recruitment of viral genome and nanohaloarchaeon D14 in previously published prokaryote and viral metagenomes from the same crystallizer pond (CR30) and other similar hypersaline systems. Metagenomic data from crystallizer CR30 studies here were obtained from Santos et al . [7] and Ghai et al . [19] Deep-Illumina sequencing data from Lake Tyrrell was from Emerson et al . [41] and Podell et al . [23] , whereas genomic data of the previously characterized Nanohaloarchaea were from Narasingarao et al . [13] BLAST+ v2.2.22 was used to recruit metagenome sequences to reference genome using the following parameters: -evalue=0.0001 –perc_identity 60 –outfmt 6. Then, BLAST hit output was parsed and plotted according to the cutoff identities and nucleotide position on viral genome. Normalization of the recruited metagenome fraction was performed according to metagenome sizes. Genome comparison of nanohaloarchaeon D14 to Candidatus Nanosalinarum J07AB56 (ref. 13 ) was performed with stand-alone BLAST version 2.2.22+ in a similar manner but using a threshold coverage and identity values of 80% in BLASTn searches in order to consider reciprocal hits. Nucleotide alignments and whole-genome alignment were performed with ClustalW and Mauve aligner [42] implemented in Geneious bioinformatics package R6.1, respectively. Genomic comparison of average nucleotide identity (ANI) and tetranucleotide frequencies between Nanohaloarchaeon D14 and Candidatus Nanosalinarum J07AB56 was carried out with the package JSpecies [43] . Dinucleotide frequencies of viral and prokaryote genomes were performed with the open programme Compseq of the The European Molecular Biology Open Software Suite 6.0.3 ( http://mobyle.pasteur.fr/cgi-bin/portal.py#forms::compseq ) with the following options: ‘-word 2 -frame 0 –reverse –ignorebz –zerocount’. Compseq uses the raw counts to estimate the ratio between expected and observed frequencies of dinucleotide signatures. These values are then used for principal component analyses using the statistical software XLSTAT (Addinsoft). For the analyses, a total of 6 genomes representing predominant hyperalophiles were considered ( Haloquadratum walsbyi, S. ruber M8, S. ruber M31, Candidatus Nanosalinarum J07AB56, Candidatus Nanosalina sp. J07AB43, host SAG D14) along with a total of 43 viral genomes previously described, 38 of which (named as ‘eHP-number’) from Garcia-Heredia and colleagues [5] and 5 viral contigs from Santos et al . [7] SNPs in the viral genome were calculated by using the bioinformatics package Geneious R6.1. P -value was calculated for all detected SNPs taking into account the probability of a sequencing error and the coverage for the position where a SNP was detected. The lower the P -value, the more likely the variation at the given position represents a SNP. For all detected SNPs, the P -values were <1 × 10 −9 . How to cite this article: Martínez-García, M. et al . Unveiling viral–host interactions within the ‘microbial dark matter’. Nat. Commun. 5:4542 doi: 10.1038/ncomms5542 (2014). Accession codes: 16S rRNA gene sequences from SAGs are deposited in the Genbank Nucleotide database with accession codes KF771589 to KF771641 . Viral and SAG D14 genome sequences are deposited in the Genbank Nucleotide database with accession codes SAMN02369554 and SAMN02369553 . The complete archaeal genome shotgun project is deposited in the GenBank Nucleotide database with accession code AYGT00000000 (the version described in this paper is version AYGT01000000 ). SAG D14 genome annotation is deposited in the RAST (Rapid Annotation using Subsystem Technology) server with accession code 6666666.48919. Raw Illumina data for single-cell and fosmid sequencing are deposited in the NCBI Bioproject database with accession code PRJNA222265 .